Confinement enhances dispersion in nanoparticle–polymer blend films Polymer nanocomposites constitute an important class of materials whose properties depend on the state of dispersion of the nanoparticles in the polymer matrix. Here we report the first observations of confinement-induced enhancement of dispersion in nanoparticle–polymer blend films. Systematic variation in the dispersion of nanoparticles with confinement for various compositions and matrix polymer chain dimensions has been observed. For fixed composition, strong reduction in glass transition temperature, T g , is observed with decreasing blend-film thickness. The enhanced dispersion occurs without altering the polymer–particle interactions and seems to be driven by enhanced matrix-chain orientation propensity and a tendency to minimize the density gradients within the matrix. This implies the existence of two different mechanisms in polymer nanocomposites, which determines their state of dispersion and glass transition. Blends of polymers and nanoparticles—polymer nanocomposites (PNC)—constitute a new class of materials exhibiting tunable and novel physical properties [1] , [2] , [3] , [4] . A major obstacle in achieving the desired properties of the blends is their state of dispersion. Extensive research has, therefore, been devoted to understand the morphological and dynamical phase diagram of such blends and the consequent role it plays in determining the physical properties of these materials [5] , [6] , [7] , [8] , [9] , [10] , [11] , [12] , [13] . On the basis of these studies, various strategies are therefore being devised to enhance the dispersibilty of various functional nanoparticles in PNCs [5] , [6] , [7] , [8] , [9] , [10] , [11] , [12] , [13] , [14] , [15] . It is believed [4] , [8] , [11] , [13] that a wetting nanoparticle–polymer interface is required for homogeneous nanoparticle dispersion in bulk PNCs. For bulk PNCs it has also been well established [5] , [6] , [8] , [11] that for dewetting grafted chain–matrix chain interface, the T g of nanoparticle–polymer blends decreases with increasing fraction of the nanoparticles, whereas T g for wetting interface increases or remains unchanged. This implies that T g and dispersion of nanoparticles cannot be tuned independently in PNCs, at least for single-component graft molecules. Recent studies, however, have also shown that dispersion and thermomechanical properties could be controlled using multicomponent grafted polymer chains [16] . On the other hand, very little is known or understood about the nature of dispersion of nanoparticles in thin polymer films [5] , [6] , [7] , [9] , [10] , [12] . This is a bit surprising since, a vast amount of research has been devoted to understanding of structure and properties of thin polymer films, especially those related to the perturbation of chain conformation [17] , [18] , [19] , [20] , [21] and glass transition due to confinement [5] , [6] , [7] , [8] , [11] , [22] , [23] , [24] , [25] . Although there is significant progress in understanding the chain conformation with confinement, some conflicting reports still exist [18] , [19] , [20] , [26] , [27] . Similarly, in the case of glass transition of thin polymer films, contradictory reports on finite size effects on T g in polymer thin films have emerged [5] , [6] , [7] , [8] , [22] , [23] , [24] . If polymer chain conformations do get perturbed due to confinement, does it affect the state of dispersion and other physical properties in thin films of PNCs? To address this fundamental question, we have probed the structure and internal morphology of polymer and PNC films of variable thickness using a combination of X-ray reflectivity (XR) and real-space imaging techniques as well as molecular dynamics (MD) simulations. We observe confinement-induced enhanced dispersion of otherwise bulk phase-segregated blends of nanoparticles and polymers. To gain insight into the mechanism responsible for enhanced dispersion of nanoparticles at a microscopic level, we used coarse-grained MD simulations, which has been widely used for PNCs [4] , [13] , [28] , [29] , [30] . We simulated uniformly grafted nanoparticles in a homopolymer matrix confined between two smooth surfaces. We find that as we decrease the distance between the two surfaces, L z , the nanoparticles tend to disperse more readily and there is a significant drop in nanoparticle density near the surfaces, as observed in the experiments, and a corresponding increase in polymer segment density. In addition, calculated bond orientational parameter for matrix polymer chains indicate considerable chain orientation at the interfaces, as observed earlier for linear polymers in confinement [31] , [32] , [33] , [34] with a finite value of this parameter being observed to persist, even in the bulk, for the thinnest films simulated. On the basis of our results, we show the effect of confinement on dispersibility, D , of nanoparticles as a function of size asymmetry f and fraction of inclusion ϕ p , which would alter the reported bulk phase behaviour [4] , [9] , [11] , [13] , [15] . As a consequence of the enhanced dispersion, we observe a reduction in T g of such blends as compared with that in the bulk at comparable nanoparticle volume fractions. Interestingly, simulations indicate that the nanoparticle–polymer interactions responsible for T g reduction do not get significantly altered with confinement. This clearly implies the existence of two different mechanisms in nanoparticle–polymer blends, which determines their dispersion and glass transition, allowing for their independent control. 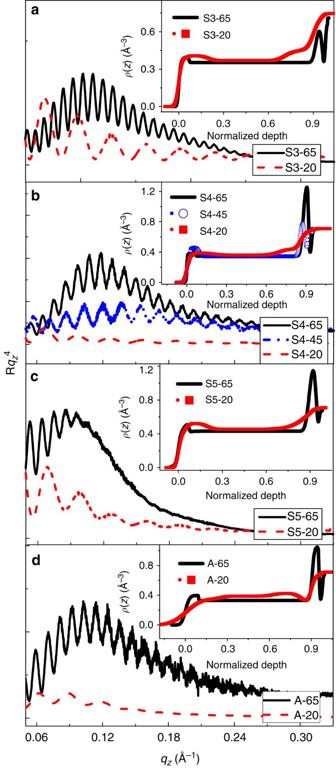Figure 1: XR profiles showing enhanced dispersion with confinement. Normalized XR profiles,versusqz, for both 65 and 20 nm films of samples S3 (a); 65, 45 and 20 nm films of samples S4 (b); 65 and 20 nm films of sample S5 (c) and sample A (d). Inset: electron density profile,ρ(z), as a function of normalized depth,z, from the air–film interface for the respective samples. In all panels, solid lines are for 65 nm while dashed lines are for 20 nm films. X-ray reflectivity Table 1 summarizes the properties of the various polymer-grafted nanoparticles (PGNPs) used in these experiments described in this manuscript. The particles have been prepared using a method described in the methods section. They have been characterized by using various methods described in the Supplementary Information ( Supplementary Fig. 1 ). Thin films of PGNPs mixed with linear polystyrene (PS) at various volume fractions, ϕ p , were prepared for thicknesses 65, 45 and 20 nm. 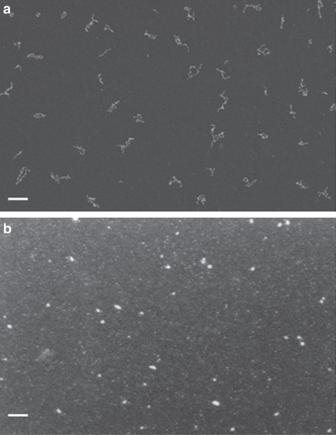Figure 2: Effect of confinement on lateral dispersion of particles. FESEM images of 65 nm (a) and 20 nm (b) films of sample S4. Effect of thickness on dispersion can be clearly seen. The bright objects are PGNPs in the background of polymer matrix. Scale bar shows 200 and 100 nm foraandb, respectively. Further details about the various samples have been specified in Table 2 . Figure 1 shows the Fresnel-normalized XR profiles of 65, 45 and 20 nm of PNC films with PGNPs of various ϕ p and f as defined in the respective panels and Table 2 . The Fresnel-normalized reflectivity allows clear visualization of the presence of modulations in the XR profile, which is indicative of density variations along the film thickness [6] , [20] , [26] . For a homogeneous thin film on a substrate, the Fresnel-normalized reflectivity consists simply of film thickness oscillations, that is, Kiessig fringes of constant or decaying amplitude depending on the magnitude of surface roughness. However, presence of density inhomogeneity or a layer of different density along the film thickness superimposes an additional modulation on the Kiessig fringes with the maximum at a wave vector q z , which is inversely proportional to the thickness of the layer. The thickness of these layers is ∼ 6 nm, which corresponds to approximately one diffuse layer of PGNPs. As can be seen in all the XR data for various 65 nm films in Fig. 1 , larger amplitude modulations are present indicative of presence of strong density inhomogeneity in these films. In Fig. 1b we also compare the XR data for 45 and 20 nm films with ϕ p =1.2% and f =0.033. Clear reduction in amplitude of the modulation with decreasing film thickness, indicative of confinement-induced density homogenization, is evident. This trend of density homogenization with confinement extends to lower ( Fig. 1a ) and higher ( Fig. 1b ) ϕ p and higher f ( Fig. 1d ). However, as f increases further, the dispersion of the PGNPs in PS films increases, leading to increased homogenization of density for such films as can be seen in Supplementary Fig. 2 . These observations are independent of the model used to extract the electron density depth profile (EDP) from respective XR data. However, to quantify these observations accurately, we extracted the respective EDP from all the XR data using detailed modelling and analysis. The corresponding extracted EDPs for the XR data are also shown in the insets in Fig. 1 . Also, refer Supplementary Note 1 and Supplementary Figs 3–7 for the details of the models used, fitted profiles and the extracted EDPs. The obtained EDPs clearly bring out the features of the distribution of PGNPs in the respective films. The EDP of 65 nm films shows clear indication of presence of high-density layers of PGNPs at the film–substrate interface, which gives rise to the modulations observed in the XR data. Reduction in film thickness leads to clear homogenization of the PGNP density and hence the enhancement of dispersion. At the highest f , the phase segregation becomes weaker to the extent that the density of these layers is much smaller compared with lowest f case ( Supplementary Fig. 7 ). The observation is along the expected lines [4] , [5] , [11] , [12] , [13] , indicating the ability to control the dispersion nanoparticles by varying f . Table 1 Properties of PGNP. Full size table Table 2 Specification of PGNP-PS composite films. Full size table Figure 1: XR profiles showing enhanced dispersion with confinement. Normalized XR profiles, versus q z , for both 65 and 20 nm films of samples S3 ( a ); 65, 45 and 20 nm films of samples S4 ( b ); 65 and 20 nm films of sample S5 ( c ) and sample A ( d ). Inset: electron density profile, ρ ( z ), as a function of normalized depth, z , from the air–film interface for the respective samples. In all panels, solid lines are for 65 nm while dashed lines are for 20 nm films. Full size image Lateral dispersion The phenomenon of confinement-induced enhancement in dispersion is further corroborated from the field emission scanning electron microscope (FESEM) images shown in Fig. 2 . While the 65 nm films show strong surface segregation and formation of domains of PGNPs, the 20 nm films are remarkably homogeneous with an enhanced bulk density of PGNPs and almost complete absence of preferred surface segregation and domain formation. Additional confirmation of confinement-induced enhanced dispersion comes from the atomic force microscopy (AFM) images of the surface morphology of these films. 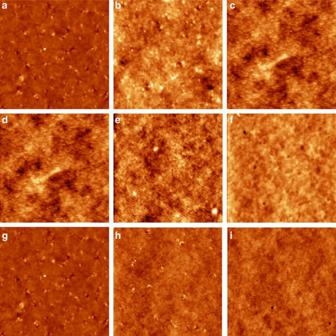Figure 3: Variation of surface morphology with confinement. AFM images of S4 samples for 65 (a), 45 (b) and 20 nm (c) films, respectively. Clear reduction in surface clustering as well as concentration of PGNPs at the surface with decreasing thickness at a fixedϕp=1.2% andf=0.033 is visible. AFM images of S4, A and C samples for both 20 (d–f) and 65 nm (g–i) thickness films, respectively. Effect of thickness and size asymmetry,f, on the lateral dispersion of PGNPs can clearly be witnessed. All the images shown are 3.0 × 3.0 μm. Figure 3 shows typical AFM surface topography images of films of various thicknesses for some of the samples specified in Table 2 . From Fig. 3a–c , we observe that surface segregation and clustering clearly reduces with decreasing film thickness for a fixed ϕ p . Similarly, for film thickness of 20 nm and ϕ p =1.2%, we observe clear enhanced dispersion of the PGNPs, with increasing f as visible in Fig. 3d–f . Further, the surface morphology of a 65-nm film for sample C ( Fig. 3i ) shows considerably reduced surface segregation and clustering as compared with that of sample S4 ( Fig. 3g ). These observations lend additional confirmation to the conclusions drawn earlier on enhanced PGNP dispersion, based on the extracted EDPs for the respective samples. The volume fraction dependence of the lateral dispersion was shown in Supplementary Figs 8–10 and discussed in Supplementary Note 2 . However, while the EDPs provide the information about the depth-dependent density profile along the film thickness, the information obtained from both AFM and FESEM is largely restricted to the surface of these films, thus nicely complementing and supporting the conclusions drawn from analysis of XR data. Figure 2: Effect of confinement on lateral dispersion of particles. FESEM images of 65 nm ( a ) and 20 nm ( b ) films of sample S4. Effect of thickness on dispersion can be clearly seen. The bright objects are PGNPs in the background of polymer matrix. Scale bar shows 200 and 100 nm for a and b , respectively. Full size image Figure 3: Variation of surface morphology with confinement. AFM images of S4 samples for 65 ( a ), 45 ( b ) and 20 nm ( c ) films, respectively. Clear reduction in surface clustering as well as concentration of PGNPs at the surface with decreasing thickness at a fixed ϕ p =1.2% and f =0.033 is visible. AFM images of S4, A and C samples for both 20 ( d – f ) and 65 nm ( g – i ) thickness films, respectively. Effect of thickness and size asymmetry, f , on the lateral dispersion of PGNPs can clearly be witnessed. All the images shown are 3.0 × 3.0 μm. Full size image Quantifying the dispersion To quantify the dispersion of PGNPs along the thickness, we have extracted their volume fraction, ϕ p , from the corresponding EDPs for the various films. The ϕ p was further subdivided in terms of bulk ϕ blk , surface ϕ sur and interface ϕ int volume fractions. The respective values must always satisfy the rule ϕ p = ϕ sur + ϕ blk + ϕ int . We further defined, ϕ seg = ϕ sur + ϕ int as the volume fraction of segregated PGNPs for respective films. 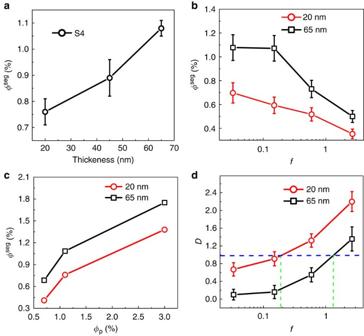Figure 4: Enhanced dispersion with confinement. ϕsegas a function of thickness (a) and size asymmetryf(b) of S-based films forϕp∼1.2%. (c)ϕsegas a function ofϕpfor two different thicknesses as identified in the panel. (d)Dversusffor a fixedϕp∼1.2% and two different thicknesses, as indicated. The error bars in the panels show the error band associated with XR modelling and analysis. Figure 4a shows ϕ seg as a function of film thickness for a fixed ϕ p and f . Clear reduction in the segregated fraction of PGNPs, ϕ seg , and hence the enhancement of bulk dispersion, with confinement, is evident. Similarly, the reduction in ϕ seg with increasing f is also evident in Fig. 4b . At fixed f , ϕ seg (20 nm) < ϕ seg (65 nm), again indicating confinement-induced enhancement of dispersion for different f . In Fig. 4c , enhanced dispersion with confinement can also be seen for various ϕ p at a fixed f . We have summarized these results in terms of the dispersibility parameter, D (= ϕ blk / ϕ seg ), in Fig. 4d . While the D for 65 nm films follows the behaviour observed in bulk PNCs [4] , [11] , the 20 nm films show enhanced dispersion, even for bulk immiscible blends of nanoparticles and polymers, indicating the possible modification of the corresponding bulk miscibility phase diagram [4] due to confinement. Coarse-grained MD simulations of melt-like PNCs confined between two parallel surfaces were performed to obtain further microscopic insight into the phenomenon of enhanced dispersion with confinement. All simulations were performed at a single ϕ p =5%, using lammps [35] . The polymers were modelled as bead-spring chains using the finite extensible nonlinear elastic potential with standard values as in [36] , with bead diameter d =1 and the nanoparticles were spheres of size D 0 =4 d . The nanoparticles were uniformly grafted with chains identical to matrix chains with a grafting density σ ∼ 1 chain/ d 2 . The degree of polymerization, N m , for matrix polymers considered in this study were 50 and 100, while that for the grafted polymers, N g , was fixed at 2. 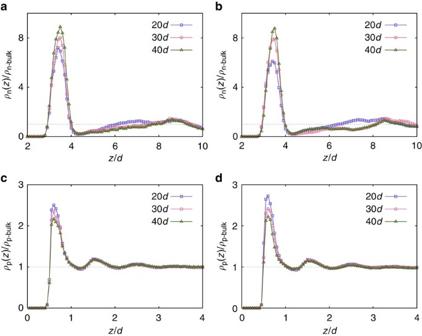Figure 5: Decreased segregation with confinement. MD simulation results of PNC confined between two parallel smooth surfaces. Normalized nanoparticle density,ρn, profile as a function of distance from the surface for increasingf, (a)f=0.02 and (b)f=0.04 for different film thicknesses indicated in respective panels as legends. The corresponding polymer density,ρp, profiles are shown inc,d, respectively. Note that the nanoparticle density at the surface decreases with confinement and the effect is more pronounced at higherf(b). Figure 5a,b shows the normalized (w.r.t. the bulk density ρ n−bulk ) density profiles, ρ n ( z ), of nanoparticles with increasing f as a function of distance from the surface for various film thickness. Since both surfaces are identical, we only show the average profiles from surface ( z =0) to a point where the densities reach their respective bulk values, ρ n−bulk . We clearly observe that the density of surface PGNP layer decreases with reduction in film thickness. As shown in Fig. 5b , the extent of this enhancement also increases with increase in effective f , which is realized in the MD simulations using a smaller matrix chain while keeping the grafted chain length fixed. This behaviour is quite consistent with our experimental observations ( c.f. Fig. 4 ). We also observe a consequent increase in matrix polymer density, ρ p ( z ), at the interface as shown in Fig. 5c,d . This indicates that, for thinner films, nanoparticles are dislodged by polymers near the surface. Figure 4: Enhanced dispersion with confinement. ϕ seg as a function of thickness ( a ) and size asymmetry f ( b ) of S-based films for ϕ p ∼ 1.2%. ( c ) ϕ seg as a function of ϕ p for two different thicknesses as identified in the panel. ( d ) D versus f for a fixed ϕ p ∼ 1.2% and two different thicknesses, as indicated. The error bars in the panels show the error band associated with XR modelling and analysis. Full size image Figure 5: Decreased segregation with confinement. MD simulation results of PNC confined between two parallel smooth surfaces. Normalized nanoparticle density, ρ n , profile as a function of distance from the surface for increasing f , ( a ) f =0.02 and ( b ) f =0.04 for different film thicknesses indicated in respective panels as legends. The corresponding polymer density, ρ p , profiles are shown in c , d , respectively. Note that the nanoparticle density at the surface decreases with confinement and the effect is more pronounced at higher f ( b ). Full size image 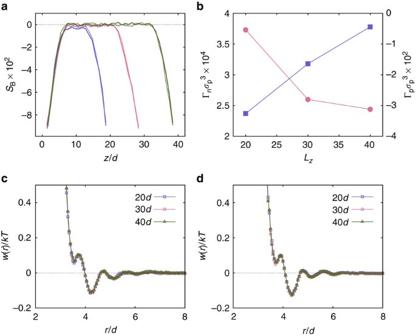Figure 6: Microscopic insight on enhanced dispersion. (a) Bond orientational parameter,Sb, as a function of depth for different thicknesses. The thickness is 20d (blue), 30d (pink) and 40d (green), respectively. Solids lines present blend systems and dotted lines present pure polymer systems. (b) Excess adsorption of polymers and nanoparticles on surface as a function of film thickness. Squares represent nanoparticles (left axis) and circles represent polymers (right axis). PGNP-matrix polymer PMF forc,f=0.02 andd,f=0.04. Interestingly, no thickness dependence is observed, although a strong repulsive barrier, signature of autophobic dewetting could be observed. Figure 6a shows the variation in bond orientational parameter S b along the depth for various thicknesses. The bond orientational order parameter was calculated as S B, i =0.5 [3‹ cos 2 θ j , z › i −1], where θ is the angle made by the bond between beads j and j −1 with z axis and ‹ …› represents the ensemble average taken over all segments of a single chain i. As expected [31] , [32] , [33] , [34] , [37] , [38] , S B becomes ∼ 0 in the bulk for the thicker films, but retains a small but noticeable value even in the bulk for the thinnest film simulated. In fact, on closer inspection ( Supplementary Fig. 11 ) it reveals that the degree of chain orientational anisotropy for the blend film is marginally higher than that of the pristine polymer film at similar thickness. To further substantiate the correlation between confinement-induced polymer chain packing alterations and PGNP dispersibility, we show in Fig. 6b the excess adsorption calculated as , where i represents the species. We note that as film thickness decreases, the excess adsorption of nanoparticles also decreases, while the excess adsorption of polymers segments increases. We would like to note here that an earlier report by Hariharan et al. [39] found similar behaviour for polymer–polymer blend films. Their results were interpreted in terms of minimization of the density gradients, created by phase segregation of one component of the blend to the interfaces, due to confinement. We feel that the mechanism for the observed confinement-induced enhanced dispersion is along similar lines. The observed reduction in agglomeration with confinement, as seen quite clearly from SEM ( Fig. 2 ) and AFM ( Fig. 3 ) images, stems from the reduction in PGNP density at the interfaces due to this tendency of density gradient minimization. Figure 6: Microscopic insight on enhanced dispersion. ( a ) Bond orientational parameter, S b , as a function of depth for different thicknesses. The thickness is 20d (blue), 30d (pink) and 40d (green), respectively. Solids lines present blend systems and dotted lines present pure polymer systems. ( b ) Excess adsorption of polymers and nanoparticles on surface as a function of film thickness. Squares represent nanoparticles (left axis) and circles represent polymers (right axis). PGNP-matrix polymer PMF for c , f =0.02 and d , f =0.04. Interestingly, no thickness dependence is observed, although a strong repulsive barrier, signature of autophobic dewetting could be observed. Full size image Does the enhanced dispersion of PGNPs indicate an effective dry–wet brush transition as far as the grafted chain–matrix chain interface is concerned? To obtain better insight into this aspect, potential of mean force (PMF) between PGNPs and polymers defined as w ( r )/ kT =− log ( g np ( r )) were calculated, as shown in Fig. 6c,d for two different values of f . Here, g np ( r ) is the two-point correlation function of particle–polymer pairs. The repulsive barrier in the effective PMF between PGNPs and polymers is due to depletion interaction-mediated autophobic dewetting of the PGNPs by the matrix chains, leading to their phase segregation as observed earlier [4] , [5] , [6] , [11] . It could be clearly seen that the particle–polymer PMF is invariant with confinement for both the f . It is thus clear that the nature of polymer–particle interaction does not depend on confinement, irrespective of the f used. Also, from the experimental point of view, given the grafting densities it is highly unlikely that the enhanced dispersion is due to the conformational transition in the grafted chains. So, both simulation and experiments point to the fact that there is no dry–wet brush transition. To illustrate the effect of enhanced dispersion on T g , we will focus on the S-series samples that have the smallest f , implying that they are the ones most likely to be affected by increase in dispersion of the particles. 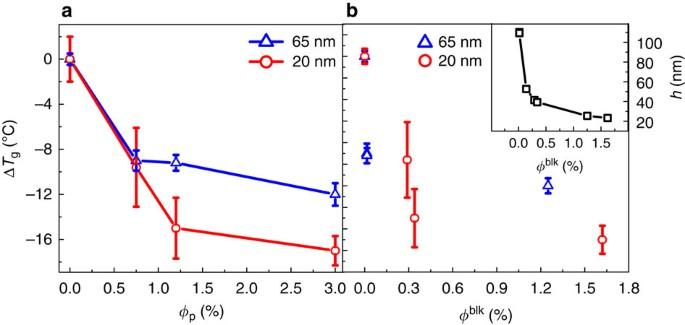Figure 7: Additional deviation ofTgof PNC films with confinement. ΔTgversusϕp(a) andϕblk(b) for S-based 20 and 65 nm films. Inset: variation of mean interparticle spacing,h, as a fucntion ofϕblk. The enhancement in ΔTgfor 20 nm films, compared with the 65 nm films at identicalϕp, can be clearly seen. Further, the extent of decrease roughly scales withϕblkand hence, mean interparticle spacing,h, establishing the link between additional bulk dispersion and change inTg. The error bars for thicker films show the thickness spread around the glass transition, while for thinner films it shows error associated with the sigmoidal fits of the data. Figure 7 shows a comparison of the relative change in T g (=Δ T g ) of PS nanoparticle composite films as compared with the respective pristine material. Data for 65 nm films have been taken from our earlier work [6] and compared with the current measurements on the 20 nm films. The T g estimates for all 20 nm films have been made using in situ temperature-dependent AFM measurements and the details are given in the Supplementary Note 3 and Supplementary Figs 12 and 13 . It is clear ( Fig. 7b ) that enhanced relative dispersion of the nanoparticles in the 20 nm films, represented by larger value of ϕ blk , leads to larger values of Δ T g at similar ϕ p , which is expected based on the nature of grafted chain–matrix chain interaction for the S-series samples. Using an approximate estimation of the mean interparticle separation, is the volume fraction of random close packing [8] ), corresponding to a particular ϕ blk value it can be seen that the Δ T g decreases with decreasing h , similar to earlier observations [8] , [11] . So how does one rationalize the observed enhancement in dispersion as well as further reduction in T g ? Simulations indicate that on the scale of chain dimensions, the polymer–polymer pair correlations, g ( r ), as shown in Supplementary Fig. 14 ( Supplementary Note 4 ), as well as the particle polymer PMF, as shown in Fig. 6c,d , is not altered. This therefore indicates that interactions at the segmental level, which essentially determine physical properties like glass transition, are not altered, significantly due to confinement. However, enhanced PGNP dispersion within the interior of the blend film increases the relative fraction of dewetting PGNP–polymer interface. Hence, the Δ T g increases further in proportion to as would be expected for a dewetting brush–polymer interface [5] , [6] , [8] , [11] . This in turn alludes to the possibility of controlling nanoparticle dispersion and T g , independently, in PNCs, under confinement. Figure 7: Additional deviation of T g of PNC films with confinement. Δ T g versus ϕ p ( a ) and ϕ blk ( b ) for S-based 20 and 65 nm films. Inset: variation of mean interparticle spacing, h , as a fucntion of ϕ blk . The enhancement in Δ T g for 20 nm films, compared with the 65 nm films at identical ϕ p , can be clearly seen. Further, the extent of decrease roughly scales with ϕ blk and hence, mean interparticle spacing, h , establishing the link between additional bulk dispersion and change in T g . The error bars for thicker films show the thickness spread around the glass transition, while for thinner films it shows error associated with the sigmoidal fits of the data. Full size image In conclusion, we report the first observation of confinement-induced enhancement of dispersion in nanoparticle–polymer blend films. We observe systematic variation in the dispersion of nanoparticles with confinement for different size asymmetry and PGNP volume fractions, which would modify their phase behaviour when compared with their bulk counter parts. Using MD simulations, the decrease in PGNP density is shown to be compensated by the corresponding increase in polymer segmental density at the surface. For one of the systems displaying enhanced dispersion, we show that its T g can also be altered from the corresponding thick-film limit. Considerable changes in polymer chain packing exemplified by surface enrichment of matrix polymer segments and considerable chain orientation primarily at the interfaces as well as in the bulk for the thinner films is observed in simulations. Our results point to the existence of confinement-induced minimization of nanoparticle density gradients within the matrix, aided by polymer chain packing and chain orientation modifications, similar to that observed earlier, while keeping the polymer–PGNP PMF invariant. This leads to simultaneous enhanced PGNP dispersion and larger reductions in blend film T g with decreasing thickness. Preparation of PGNP Here we discuss the synthesis of polymer-grafted gold nanoparticles. We used the reduction and in situ grafting-to method first described by Lennox and coworkers [40] . Freshly distilled tetrahydrofuran (THF) is used as a solvent medium, and all the reactants were dissolved in THF. A typical synthesis will consist of mixing thiol-terminated PS and chloroauric acid (HAuCl 4 .3H 2 O) and made to stirr for half an hour. The reduction of chloroauric acid is started with the addition of 0.5 M super hydride (lithium triethyl borohydride) at once, with which the solution turns dark brownish pink. The total reaction is carried out in dark environment. The mixture is stirred for a couple of more hours, and then ethanol is poured (1:3) in, to selectively precipitate the particles. The solution is then centrifuged at 5,000 r.p.m. for 5 min to seperate out the particles. The supernatant was discarded, the nanoparticles were redissolved in THF to which ethanol is added and then centrifuging process was repeated for 3–5 times, so that all the ungrafted free chains could be removed. The different physical properties of PGNPs were summarized in Table 1 . The grafting densities were measured using the combination of thermogravimetric analysis (weight ratio of graft chains to the gold core) and the size obtained from transmission electron mcroscopy, using standard methods described earlier [6] , [7] , [40] . Preparation of PNC films The PGNPs as obtained were stirred in toluene for a day, and atactic PS (MW-20 and 90 kg mol −1 ) were also stirred in toluene for a day. These pristine polymer and particle solutions were mixed in appropriate ratios to obtain samples as defined in Table 2 . These mixtures were stirred for ∼ 24 h, to ensure homogenization of the samples. These solutions were then used to spin cast PNC films of required thickness. Before spin casting, the silicon wafers (2 inch Si ‹ 100› wafer bought from Vin Karola, USA) were first cut into 10 × 10 mm pieces and were then cleaned using freshly prepared Piranha solution (70:30 mixture of sulphuric acid and hydrogen peroxide, respectively). The substrates were kept in the freshly prepared Piranha solution for 10 min and then rinsed with de-ionized water (18.2 MΩ resistance) for few times. These substrates were then used to spin cast the solutions prepared. The films as prepared were annealed at 150 °C ( T g of PS 90 kg mol −1 is 106 °C) for 12 h. This high-temperature annealing removes the trapped solvent and also ensures an equilibrium dispersion of particles. X-ray reflectivity The dispersion of the particles along the depth were quantified using specular XR. XR is an invasive, non-destructive method, where the reflected intensity from the sample is proportional to the density gradient along the thickness of the film. This very nature of reflectivity’s dependency could be used to find the surface/interface phase segregations, without modelling the data (as discussed with the normalized reflectivity profiles in Fig. 1 ). XR measurements were performed with both synchrotron radiation (BL 18B in Photon Factory synchrotron, Tsukuba, Japan) at an incident X-ray energy of 12 keV as well as with a lab source (D8 Discover, Bruker, Germany) at 8 keV. The electron density profile, EDP ( ρ ( z )), of the various films were extracted from the measured XR as a function of the perpendicular wave vector transfer, q z [6] , using IGOR PRO—MOTOFIT [41] . All the data discussed in this article were modelled with a three-slab model whose descriptions and more details are given in the Supplementary Information . Field emission scanning electron microscopy FESEM (Ultra, Carl Zeiss, Germany) is used to find the lateral dispersion of the particles. FESEM is used in in lens mode at a working distance of 2–3 mm with an operating voltage of 8–10 keV. As it is known that with AFM we could only see surface topography, whereas with the help of penetration depth of electrons in FESEM, we could see dispersion of particles in slight interior of the films as well. With the depth of the features increasing, the contrast goes down. By looking at the contrast we could clearly say the lateral dispersion in the surface and dispersion in the interior of the film (penetration depth depends on parameters like operating voltage, dielectric constant of the sample, working distance, and so on). AFM and temperature-dependent atomic force spectroscopy Surface topography of the samples was imaged using AFM (NT-MDT, Russia) in contact mode. Cantilevers with a force constant of 0.03–0.2 N m −1 and radius of curvature ≤15 nm were used for imaging. The images were collected at a scanning velocity of 3–5 μm s −1 and at a minimum normal force (to avoid dragging of the tip on the sample) as determined from force-displacement curve. Also, it is well known that the polymer films through the glass transition temperature, T g , will change from a hard and brittle-like to soft and fragile. Temperature-dependent AFM-based force-distance spectroscopy has been used to find the mechanical properties of the film for a series of temperatures. The methodology used for collecting the data is as follows: the samples were kept in an environment-controlled sample chamber and the chamber is purged with nitrogen gas at a rate of 40 ml min −1 . The sample was heated at a rate of 1 °C min −1 and the force-displacement curve is measured at every 3 °C interval. Force-distance spectroscopy is a widely used [42] , [43] technique that senses the local forces on the sample with a spatial resolution of the order of few tens of nm. Force-displacement curve is a plot between the tip–sample interaction force ( F ) and the displacement of the sample towards tip ( Z ). The slope gives a measure of the elastic modulus of the sample [42] , [43] . The re-trace or trace parts of the force-distance curves were fitted with a straight line and the slopes are extracted at each temperature. Ten to fifteen measurements at each temperature is made to get a statistically averaged data. Refer Supplementary Figs 12 and 13 for the data and extraction of T g respectively. Coarse-grained molecular dynamic simulations The PNC systems considered in this study were made of bead-spring polymer chains and uniformly grafted spherical nanoparticles with a total packing fraction (in reduced units, d and D 0 are the sizes of polymer segment and nanoparticles, respectively). To study the effect of confinement on these systems, the PNCs were simulated between two infinitely long smooth surfaces perpendicular to the z axis. Systems with three different distances between the surfaces ( L z =20 d , 30 d and 40 d ) were considered. Periodic boundary conditions were enforced in x and y directions. The pair-wise interactions between all particles in the system were defined using a shifted Lennard–Jones (LJ) potential of the form, where, ε is the well-depth, r is the distance between two particles, Δ is the shift parameter and r c is the cutoff distance beyond which the potential is truncated and shifted to 0. This form of potential was chosen such that the non-bonded interactions for all particles as a function of distance from the particle surface are the same, regardless of particle diameter. Thus, the shift parameters Δ pp =Δ gg =Δ pg =0, while Δ nn = D 0 − d , Δ pn =( D 0 − d )/2 and Δ gn =( D 0 − d )/2 where, p, g and n represent matrix polymers, grafted polymers and nanoparticles, respectively. How to cite this article: Chandran, S. et al. Confinement enhances dispersion in nanoparticle–polymer blend films. Nat. Commun. 5:3697 doi: 10.1038/ncomms4697 (2014).